Theoretical models of nonlinear effects in two-component cooperative supramolecular copolymerizations The understanding of multi-component mixtures of self-assembling molecules under thermodynamic equilibrium can only be advanced by a combined experimental and theoretical approach. In such systems, small differences in association energy between the various components can be significantly amplified at the supramolecular level via intricate nonlinear effects. Here we report a theoretical investigation of two-component, self-assembling systems in order to rationalize chiral amplification in cooperative supramolecular copolymerizations. Unlike previous models based on theories developed for covalent polymers, the models presented here take into account the equilibrium between the monomer pool and supramolecular polymers, and the cooperative growth of the latter. Using two distinct methodologies, that is, solving mass-balance equations and stochastic simulation, we show that monomer exchange accounts for numerous unexplained observations in chiral amplification in supramolecular copolymerization. In analogy with asymmetric catalysis, amplification of chirality in supramolecular polymers results in an asymmetric depletion of the enantiomerically related monomer pool. A detailed understanding of the self-assembly of molecules in multi-component mixtures resulting in supramolecular architectures of well-defined composition is critical when trying to rationalize their application in different functions like optoelectronic devices [1] , [2] , catalysis [3] , [4] and biomimetic materials [5] , [6] . Although the physical basis of self-assembly under thermodynamical control of single-component [7] , [8] , [9] , [10] , [11] , [12] , [13] , [14] systems is well understood, chemists have only recently started to formulate models and concepts that capture self-assembly of molecules in multi-component mixtures [15] , [16] , [17] , [18] , [19] , [20] , [21] , [22] . These multi-component systems are characterized by the presence of a network of coupled association equilibria, which can lead to unexpected solution compositions, as small differences in association energies are amplified at the level of the supramolecular assemblies [19] , [22] , [23] , [24] . The theoretical description of self-assembly in multi-component mixtures has been mainly applied to discrete supramolecular assemblies [15] , [16] , [17] , [18] , [19] , [20] . However, often one or more of the components in the mixture are able to undergo supramolecular polymerization, which leads to an infinite number of possible molecular complexes. As such, the analysis of such mixtures is a challenging task [22] . Here, we formulate a general model for cooperative supramolecular copolymerization in a two-component mixture, and apply it to rationalize chiral amplification in helical supramolecular polymers. Amplification of chirality in helical covalent and supramolecular polymers can occur via the sergeants-and-soldiers or the majority-rules principle as first proposed by Green et al . [25] , [26] for the case of covalent, helical polyisocyanates. In the sergeants-and-soldiers principle, (supramolecular) copolymerization of an achiral monomer with a small amount of homochiral monomer leads to a strong bias towards the macromolecular helicity corresponding to the chiral enantiomer. In the majority-rules principle, (supramolecular) copolymerization in mixtures of two enantiomers using a slight excess of one enantiomer leads to a strong bias towards the macromolecular helicity corresponding to the major enantiomer. We have recently reported temperature-dependent sergeants-and-soldiers [27] , [28] and majority-rules [28] , [29] titrations in mixtures of chiral and achiral N , N ′, N ″-trialkylbenzene-1,3,5-tricarboxamides (BTAs) that self-assemble into helical, dynamic supramolecular polymers via three-fold, cooperative hydrogen bonding ( Fig. 1 ) [30] , [31] , [32] , [33] , [34] . In the absence of chiral centres at the periphery, the helical supramolecular polymers form by definition as a racemic mixture of P and M enantiomers. However, when chiral components are used, the P and M isomers have a diastereomeric relationship and consequently have unequal energy. The temperature-dependent chiral amplification in mixtures of self-assembling chiral and achiral BTAs was probed using circular dichroism (CD) spectroscopy and analysed using modified [35] , [36] 1D Ising models adapted from the theory of helical, covalent polymers. As these models have originally been developed for covalent, irreversible polymerizations, they do not consider the full complexity of all equilibria present in the two-component mixture, such as the equilibrium between the monomer pool and aggregates, and the strong cooperative growth of the assemblies. 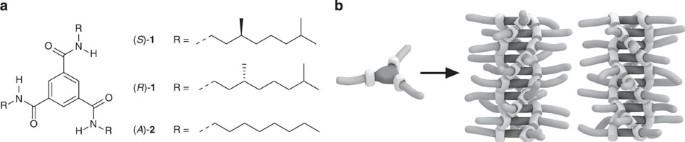Figure 1: Chiral BTA self-assembly. (a) Structures ofN,N′,N″-trialkyl-benzene-1,3,5-tricarboxamides (BTAs) equipped with achiral, (R)-chiral and (S)-chiral aliphatic side chains. (b) Schematic picture of the cooperative supramolecular copolymerization into supramolecular polymers with two types of helicity (PandM). In the absence of chiral centres at the periphery, the helical supramolecular polymers form by definition a racemic mixture ofPandMenantiomers. However, when chiral components are used, thePandMhelices have a diastereomeric relation and consequently have unequal energy. Figure 1: Chiral BTA self-assembly. ( a ) Structures of N , N ′, N ″-trialkyl-benzene-1,3,5-tricarboxamides (BTAs) equipped with achiral, ( R )-chiral and ( S )-chiral aliphatic side chains. ( b ) Schematic picture of the cooperative supramolecular copolymerization into supramolecular polymers with two types of helicity ( P and M ). In the absence of chiral centres at the periphery, the helical supramolecular polymers form by definition a racemic mixture of P and M enantiomers. However, when chiral components are used, the P and M helices have a diastereomeric relation and consequently have unequal energy. Full size image Here we present two novel methodologies to describe chiral amplification in two-component, self-assembling systems that take into account the coupling between the cooperative growth of the supramolecular polymer and the monomer pool. Both methodologies are based on a common reaction scheme in which supramolecular copolymerization is described as a sequence of stepwise monomer addition and dissociation events. In the first approach, the equilibrium concentrations of all species are obtained by solving the mass-balance equations for the two monomer types. In the second approach, a stochastic simulation algorithm (SSA) based on the Gillespie method is used to obtain these equilibrium concentrations. Both methodologies can be applied to model chiral amplification either arising via the sergeants-and-soldiers or the majority-rules principle. By illustrating the mass-balance-based approach on the majority-rules principle, we present evidence for the dominant effect of monomer exchange on chiral amplification in supramolecular polymers ultimately leading to an asymmetric depletion of the enantiomerically related monomer pool. By applying the SSA to the sergeants-and-soldiers principle, we rationalize previously unexplained features of CD titration experiments obtained by mixing chiral and achiral BTAs. Although computationally more demanding, the stochastic simulations provide detailed insight into the chiral amplification kinetics, which can be visualized as movies. Such movies greatly increase the understanding of association phenomena in complex and multi-component mixtures of self-assembling molecules that are continuously in exchange. Cooperative supramolecular copolymerization Consider the simplest model possible for a general supramolecular polymerization of a single monomer (X). The only reactions allowed are stepwise additions and dissociations of single monomers from one end of the supramolecular polymer. The corresponding set of reaction equations is given by where X i denotes the polymers of length i , X 1 =X denotes the monomers, and k i + (M −1 s −1 ) and k i − (s −1 ) are the rate constants of the forward and backward reactions, that is, for the addition or removal of a monomer unit. The equilibrium constant for this reaction is given by . Depending on the evolution of K i as a function of chain length ( i ), the supramolecular polymerization can be classified either as isodesmic ( K 1 = K 2 = ... = K iso ) or as cooperative ( K 1 = K 2 =...= K n −1 < K n = K n +1 = ... = K elo ), where n is the nucleus size. The equilibrium constants are related to the standard Gibbs free energy difference by where is the standard Gibbs free energy increment for the addition of a monomer to a polymeric chain of length i , R is the gas constant and T the temperature. The change in standard Gibbs free energy can be calculated from the enthalpy and entropy increment by the relation Our model for chiral amplification in two-component, cooperative supramolecular polymerizations generalizes this approach in the sense that every individual monomer X can be of two different types, and that supramolecular polymers of two types of helicity ( P - or M -type) can be assembled. As the supramolecular polymerization of BTAs occurs via a cooperative mechanism, the reactions for each polymer type are divided in a nucleation and an elongation phase in which we have assumed a nucleus size of 2. This assumption is reinforced by previous gas-phase DFT calculations [34] , and the notion that the melting curves obtained using CD and UV–Vis spectroscopy are identical [14] . The distinction between P - or M -type helical aggregates is made at the nucleus formation stage. Once a nucleus of length two is formed, the helicity of the aggregates is maintained in subsequent monomer addition and dissociation reactions until the aggregate is completely broken down. 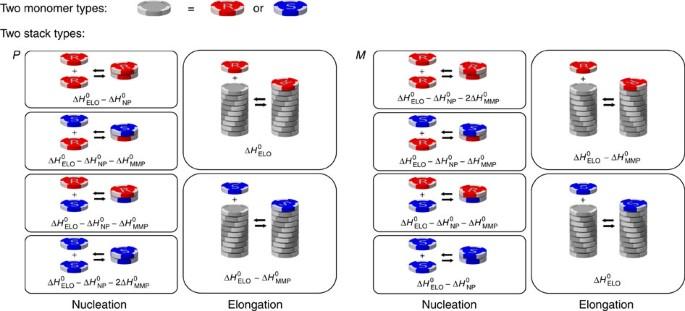Figure 2: Majority-rules reactions. Possible reactions and corresponding enthalpy differences in the majority-rules model, where (R)-chiral (red) and (S)-chiral (blue) monomers reversibly associate into helical supramolecular copolymers with opposite helicity (PandMtype). Possible reactions are the formation ofP- orM-type dimers, the dissociation of existing dimmers, and the addition or dissociation of monomeric units to/from existing oligomers/polymers. The addition of chiral monomers to supramolecular polymers having their preferred helicity (that is,R-chiral monomers prefer to associate withP-type helical aggregates whileS-chiral monomers prefer to associate withM-type helical aggregates) is described by an elongation enthalpyand entropy ΔS0. The addition of chiral monomers to supramolecular polymers with the wrong handedness (that is, association of anR-chiral monomer to anM-type helical supramolecular polymer and association of anS-chiral monomer to aP-type helical supramolecular polymer) is penalized by a mismatch enthalpy. Nucleation of a new homo or heterochiral dimer of any type is penalized by a nucleation penaltyand an additionalfor each monomer of the wrong chirality with respect to the aggregate helicity. For the majority-rules system, we consider two enantiomerically related monomers in which each monomer addition occurs with an entropy difference Δ S 0 , while the enthalpy difference depends on the reaction type as shown in Figure 2 . The addition of monomers to their preferred aggregate type is described by a favourable elongation enthalpy, [36] . For addition of monomers to their unpreferred aggregate helicity, this elongation enthalpy is reduced by a mismatch enthalpy . In the nucleation phase, the favourable enthalpy release, , is penalized by a nucleation penalty, , and the additional mismatch penalty for each monomer of the wrong chirality. Figure 2: Majority-rules reactions. Possible reactions and corresponding enthalpy differences in the majority-rules model, where ( R )-chiral (red) and ( S )-chiral (blue) monomers reversibly associate into helical supramolecular copolymers with opposite helicity ( P and M type). Possible reactions are the formation of P - or M -type dimers, the dissociation of existing dimmers, and the addition or dissociation of monomeric units to/from existing oligomers/polymers. The addition of chiral monomers to supramolecular polymers having their preferred helicity (that is, R -chiral monomers prefer to associate with P -type helical aggregates while S -chiral monomers prefer to associate with M -type helical aggregates) is described by an elongation enthalpy and entropy Δ S 0 . The addition of chiral monomers to supramolecular polymers with the wrong handedness (that is, association of an R -chiral monomer to an M -type helical supramolecular polymer and association of an S -chiral monomer to a P -type helical supramolecular polymer) is penalized by a mismatch enthalpy . Nucleation of a new homo or heterochiral dimer of any type is penalized by a nucleation penalty and an additional for each monomer of the wrong chirality with respect to the aggregate helicity. 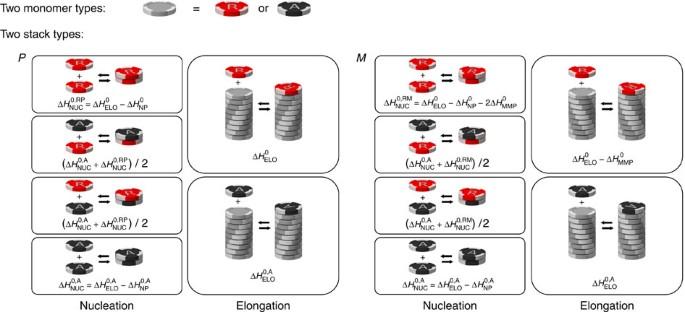Figure 3: Sergeants-and-soldiers reactions. Possible reactions and corresponding enthalpy differences in the sergeants-and-soldiers model, where (R)-chiral (red) and achiral (black) monomers reversibly associate into helical supramolecular copolymers with opposite helicity (PandMtype). Possible reactions are the same as in the majority-rules model (Fig. 2), only some of the enthalpy and entropy changes are different. The formation of homochiral dimers and elongation with chiral monomers are equal to the majority-rules model and described byand ΔS0. The addition of an achiral monomer to bothP-type andM-type aggregates during the elongation phase is described by an elongation enthalpyand entropy ΔS0,A, thus being independent on the handedness of the aggregate. Formation of aP- orM-type achiral homodimer occurs, independent on the handedness of the dimer, with an enthalpy releasewhereis the achiral nucleation penalty. Finally, the enthalpy and entropy increments of the heterodimers are, analogous to the majority-rules case, the averages of the enthalpy and entropy increments of the corresponding homodimers. Full size image For the sergeants-and-soldiers system, shown in Figure 3 , the ( R )-chiral monomers behave the same as for majority-rules, whereas the addition of achiral monomers ( A ) is described by an entropy difference Δ S 0,A elongation enthalpy , and nucleation penalty , independent of the helicity. Finally, the entropy and enthalpy increments of the heterodimers are, analogous to the majority-rules case, the averages of the increments for corresponding homodimers. In contrast to chiral-amplification models that have been constructed for covalent polymers [26] , [37] , our model does not incorporate a helix reversal penalty. Such a helix reversal penalty represents a free-energy penalty of a helix reversal along the covalent chain. We believe that such helix reversals do not exist in self-assembled supramolecular polymers, as such high-energy structures can easily be avoided by dissociation of monomers back into solution. Figure 3: Sergeants-and-soldiers reactions. Possible reactions and corresponding enthalpy differences in the sergeants-and-soldiers model, where ( R )-chiral (red) and achiral (black) monomers reversibly associate into helical supramolecular copolymers with opposite helicity ( P and M type). Possible reactions are the same as in the majority-rules model ( Fig. 2 ), only some of the enthalpy and entropy changes are different. The formation of homochiral dimers and elongation with chiral monomers are equal to the majority-rules model and described by and Δ S 0 . The addition of an achiral monomer to both P -type and M -type aggregates during the elongation phase is described by an elongation enthalpy and entropy Δ S 0,A , thus being independent on the handedness of the aggregate. Formation of a P - or M -type achiral homodimer occurs, independent on the handedness of the dimer, with an enthalpy release where is the achiral nucleation penalty. Finally, the enthalpy and entropy increments of the heterodimers are, analogous to the majority-rules case, the averages of the enthalpy and entropy increments of the corresponding homodimers. 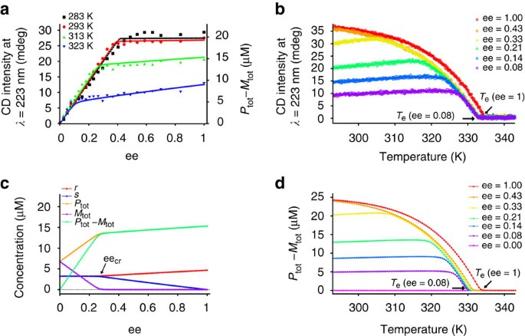Figure 4: Majority-rules data and model results. (a) CD intensity at 223 nm versus the ee for four different temperatures obtained by addition of aliquots of the (S) enantiomer of1to a solution of the (R) enantiomer at a total constant concentration of 2.0×10−5M in MCH (large symbols)28. The solid lines correspond to the calculated excess helicity (Ptot−Mtot), defined as the concentration difference of BTA molecules belonging toP- andM-type supramolecular polymers obtained using the majority-rules model with thermodynamic constants as given in the Methods and a mismatch enthalpy of −2.1 kJ mol−1. (b) Measured temperature-dependent CD intensity at 223 nm for (S)-1:(R)-1mixtures having different ee values (ctot=2.5×10−5M in MCH)28. (c) Computed speciation plot at 313 K: monomer concentrations (rands), concentration of BTA molecules belonging toP-type (Ptot) andM-type (Mtot) supramolecular polymers and their difference (Ptot−Mtot) as a function of the ee andctot=2.0×10−5M. (d) Calculated temperature-dependent helical excess (Ptot−Mtot) for several values of the ee using the same thermodynamic parameters as ina, but atctot=2.5×10−5M. Full size image The majority-rules principle The large symbols in Figure 4a show the previously reported CD intensity monitored at 223 nm as a function of the enantiomeric excess (ee) obtained by addition of aliquots of the ( S )-enantiomer of 1 to a solution of the ( R )-enantiomer at a total constant concentration of 2.0×10 −5 M in methylcyclohexane (MCH) at several temperatures [28] . As expected for a two-component system in which chiral amplification evolves via the majority-rules principle, a nonlinear dependence of the CD effect as a function of the ee is observed at all temperatures. The nonlinearity is expressed by a strong increase in the CD effect at low ee values (regime I) and a weaker increase in the CD effect at high ee values (regime II). The weaker increase in the CD effect at high ee values is especially notable at higher temperatures. Figure 4b displays the temperature-dependent CD data obtained for the ( S )- 1 :( R )- 1 mixtures in MCH [28] . In all cases, a clear elongation temperature ( T e ) is observed, characteristic for the cooperative growth of the supramolecular polymers [13] , [14] . Apart of being dependent on the total concentration ( Supplementary Fig. S1 ), the data in Figure 4b show a decrease of T e for mixtures in which the ee is lower than 1. Remarkably, for low ee values, a plateau in the CD intensity is reached that slightly decreases upon lowering the temperature. Figure 4: Majority-rules data and model results. ( a ) CD intensity at 223 nm versus the ee for four different temperatures obtained by addition of aliquots of the ( S ) enantiomer of 1 to a solution of the ( R ) enantiomer at a total constant concentration of 2.0×10 −5 M in MCH (large symbols) [28] . The solid lines correspond to the calculated excess helicity ( P tot − M tot ), defined as the concentration difference of BTA molecules belonging to P - and M -type supramolecular polymers obtained using the majority-rules model with thermodynamic constants as given in the Methods and a mismatch enthalpy of −2.1 kJ mol −1 . ( b ) Measured temperature-dependent CD intensity at 223 nm for ( S )- 1 :( R )- 1 mixtures having different ee values ( c tot =2.5×10 −5 M in MCH) [28] . ( c ) Computed speciation plot at 313 K: monomer concentrations ( r and s ), concentration of BTA molecules belonging to P -type ( P tot ) and M -type ( M tot ) supramolecular polymers and their difference ( P tot − M tot ) as a function of the ee and c tot =2.0×10 −5 M. ( d ) Calculated temperature-dependent helical excess ( P tot − M tot ) for several values of the ee using the same thermodynamic parameters as in a , but at c tot =2.5×10 −5 M. Full size image The molar concentrations of all species can be obtained by solving the mass-balance equations for the two components. For a nucleus size of two, the corresponding model is a generalization of the K 2 -K model for single-component supramolecular polymerizations as previously analysed by various authors [9] , [12] , [14] , [38] . The temperature-dependent equilibrium constants in the elongation phase are which describe equilibrium between free chiral monomers and aggregates having a preferred and non-preferred helical sense, respectively. Cooperativity is introduced by energetically disfavouring all dimerization steps using a dimensionless nucleation factor, σ The total concentration of ( R )- 1 in P -type aggregates can be derived by applying the principle of detailed balance (Methods section), which leads to where and r =[( R )- 1 ] and s =[( S )- 1 ] are the free-monomer concentrations. Analogously, the total concentration of ( R )- 1 in M -type polymers can be expressed as where Mass-balance analysis now links the total concentration ( R )- 1 ( r tot ) to the free monomer concentrations of ( R )- 1 ( r ) and ( S )- 1 ( s ) and the equilibrium constants K E1 , K E2 and nucleation factor σ according to In a similar fashion, the mass-balance condition of ( S )-chiral material leads to Equations (9) and (10) together constitute a system of two nonlinear equations from which the free monomer concentrations r and s can be solved numerically. From the obtained values, the total concentration of BTA molecules in P - and M -type aggregates ( P tot and M tot ) can be calculated (Methods section). The solid lines in Figure 4a show the calculated excess helical sense ( P tot − M tot ) as a function of ee obtained using the appropriate thermodynamic constants for the single-component systems (Methods) and a temperature-independent mismatch penalty, , of −2.1 kJ mol −1 . The calculations clearly show that, for all temperatures considered, the model is able to capture the nonlinear increase in excess helicity as the ee increases. In contrast to previously reported majority-rules models, which are based on theories developed for covalent polymers, this model correctly predicts that the CD intensity slowly increases at high ee values towards the limiting CD intensity corresponding to homochiral aggregates. To rationalize the origin of the nonlinear effects, we analysed the speciation plots in detail. Figure 4c displays the calculated concentration of chiral BTA monomers present in P - and M -type assemblies together with the free monomer concentrations, r and s , as a function of the ee for a temperature of 313 K. For ee values smaller than a critical value (ee cr ), the free monomer concentrations r and s are almost equal to each other and approximately constant. In the same ee range, the total material in P -type supramolecular polymers ( P tot ) grows linearly as a function of ee while the total material in M -type assemblies ( M tot ) decreases linearly until it is approximately zero at ee cr . Consequently, the CD effect, which is proportional to P tot − M tot , increases linearly in this regime. Intriguingly, for ee values larger than ee cr , the free monomer concentrations r and s start to deviate from each other. The slow increase in excess helicity ( P tot − M tot ) in the high ee regime (>ee cr ) is caused by the fact that the free monomer concentration s decreases faster than the free monomer concentration r increases in this regime. At lower temperatures, the monomer concentrations are much lower, thus making the slope in the CD intensity almost zero. The critical value of ee is given by see the Methods section for an explicit derivation. Note that the separation into two regimes is typical for cooperative copolymerizations and is absent for isodesmic supramolecular copolymerizations ( Supplementary Fig. S2a ). 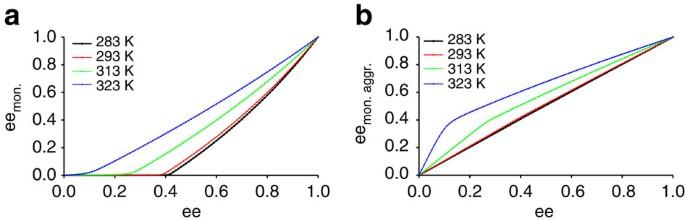Figure 5: Nonlinear effects. (a) Nonlinear behaviour of ee of the monomer pool (eemon) as a function of the ee. A strong negative nonlinear effect is observed at low temperatures indicating an asymmetric depletion of the monomer pool. (b) Nonlinear behaviour of ee of monomers present in aggregates (eemon. aggr.) computed as a function of ee. A strong positive nonlinear effect is observed at high temperatures indicating an enantiomeric enrichment of monomers present in aggregates with respect to the original solution. The thermodynamic parameters and concentration are equivalent toFigure 4a. Figure 5a plots the calculated ee of the monomer pool as a function of the total ee for all temperatures. For low temperatures, the graphs reveal a strong negative nonlinear effect indicating that the enantiomerically related monomer pool becomes asymmetrically depleted as a result of aggregation. Similar asymmetric depletion effects have been reported by Kagan and co-workers to rationalize nonlinear effects in asymmetric catalysis [39] , [40] . The asymmetric depletion of the monomer pool corresponds with an enantiomeric enrichment of monomers present in helical aggregates ( Fig. 5b ), as evidenced by a strong positive nonlinear effect, which is most notable at higher temperatures where the monomer concentrations are higher and which is again almost absent in case of isodesmic polymerization ( Supplementary Fig. S2b ). Figure 5: Nonlinear effects. ( a ) Nonlinear behaviour of ee of the monomer pool (ee mon ) as a function of the ee. A strong negative nonlinear effect is observed at low temperatures indicating an asymmetric depletion of the monomer pool. ( b ) Nonlinear behaviour of ee of monomers present in aggregates (ee mon. aggr. ) computed as a function of ee. A strong positive nonlinear effect is observed at high temperatures indicating an enantiomeric enrichment of monomers present in aggregates with respect to the original solution. The thermodynamic parameters and concentration are equivalent to Figure 4a . Full size image Given the good agreement between the model and the experimental titrations, we next sought to understand the decrease in T e as observed in the experimental melting curves ( Fig. 4b ). Figure 4d displays the calculated melting curves using the same ee values and previously described thermodynamic parameters. Indeed, the calculations correctly predict the decrease of T e as the ee value becomes smaller than 1. The decrease of T e reflects the lower stability of hetero-aggregates consisting of ( S )- 1 and ( R )- 1 caused by the unfavourable mismatch enthalpy. Moreover, the observed slightly inclined plateau in the CD intensity at lower temperatures can be rationalized by the stronger growth of M -type helical assemblies compared with P -type assemblies as the temperature is lowered ( Supplementary Fig. S3 ). 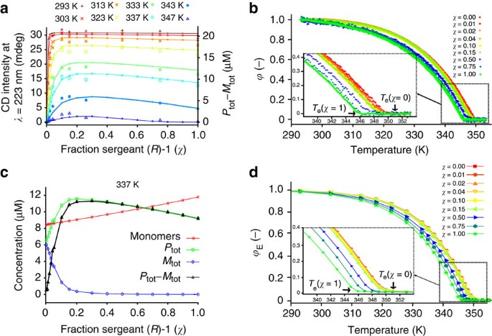Figure 6: Sergeants-and-soldiers data and model results. (a) CD intensity atλ=223 nm versus fraction of 'sergeant' (R)-1(χ), for eight different temperatures at a total concentration of (R)-1+(A)-2of 2.1×10−5M in heptane. The large symbols represent the measured CD intensities at 223 nm while the small symbols connected by broken lines correspond to the excess helical sense, defined as the concentration difference of material present inP- andM-type supramolecular polymers, as calculated by the SSA. (b) Normalized degree of aggregation (ϕ) as a function of temperature27obtained by UV–Vis spectroscopy for various mole fractions of 'sergeant' (R)-1. (c) Speciation plot at 337 K: total monomer concentration, concentration of BTA molecules belonging toP- andM-type supramolecular polymers and their difference (Ptot−Mtot) as a function of the mole fraction 'sergeant'. (d) Simulated normalized melting curves for various mole fractions of sergeant (R)-1. Due to the lowerTeof pure (R)-1supramolecular homopolymers compared with pure achiral supramolecular homopolymers, addition of aliquots of (R)-1to a solution of (A)-2results in a decrease of theTeof supramolecular heteropolymers consisting of (R)-1and (A)-2. The fraction of aggregation at equilibrium,ϕE, is calculated as (ctot−[monomers])/ctot, where [monomers] represents the total concentration of chiral and achiral monomers. The sergeants-and-soldiers principle Figure 6a (left axis) shows the CD intensity at 223 nm as a function of added 'sergeant' obtained by titrations at several temperatures in which the fraction, χ , of 'sergeant' ( R )- 1 was varied while keeping the total concentration of ( R )- 1 and ( A )- 2 constant (2.1×10 −5 M, heptane) [27] . At the lowest temperature, addition of 4% of 'sergeant' results in an excess helical sense corresponding to assemblies consisting exclusively of ( R )- 1 , a clear sign that the sergeants-and-soldiers principle is operative. Theory and experiments concerning the sergeants-and-soldiers effect in covalent polymers have shown that a larger chiral bias always results in an increase in helical sense control [25] , in contrast to majority-rules where larger chiral bias leads to a decrease in helical sense control [41] . For helical supramolecular polymers, we observe the same effect for low fractions of sergeant. However, counterintuitively, a larger chiral bias ( χ >15%) results, as especially notable at higher temperatures, in a decrease in CD intensity, suggesting either a decrease in helical sense control or a decrease in helical order. Figure 6b displays the previously reported [27] temperature-dependent CD curves obtained for the ( A )- 2 :( R )- 1 mixtures in heptane. Again, all melting curves are characterized by a well-defined T e , which shifts to lower temperatures as χ increases. Figure 6: Sergeants-and-soldiers data and model results. ( a ) CD intensity at λ =223 nm versus fraction of 'sergeant' ( R )- 1 ( χ ), for eight different temperatures at a total concentration of ( R )- 1 +( A )- 2 of 2.1×10 −5 M in heptane. The large symbols represent the measured CD intensities at 223 nm while the small symbols connected by broken lines correspond to the excess helical sense, defined as the concentration difference of material present in P - and M -type supramolecular polymers, as calculated by the SSA. ( b ) Normalized degree of aggregation ( ϕ ) as a function of temperature [27] obtained by UV–Vis spectroscopy for various mole fractions of 'sergeant' ( R )- 1 . ( c ) Speciation plot at 337 K: total monomer concentration, concentration of BTA molecules belonging to P - and M -type supramolecular polymers and their difference ( P tot − M tot ) as a function of the mole fraction 'sergeant'. ( d ) Simulated normalized melting curves for various mole fractions of sergeant ( R )- 1 . Due to the lower T e of pure ( R )- 1 supramolecular homopolymers compared with pure achiral supramolecular homopolymers, addition of aliquots of ( R )- 1 to a solution of ( A )- 2 results in a decrease of the T e of supramolecular heteropolymers consisting of ( R )- 1 and ( A )- 2 . The fraction of aggregation at equilibrium, ϕ E , is calculated as ( c tot −[monomers])/ c tot , where [monomers] represents the total concentration of chiral and achiral monomers. Full size image We next sought to understand these features in detail. In principle, the time-dependent molar concentration of all species can be obtained by numerical integration of the nonlinear reaction-rate equations as previously analysed for single-component systems [42] , [43] , [44] . However, for systems with multiple components, this approach is no longer feasible as the number of differential equations increases exponentially. Hence, we present an alternative approach using kinetic Monte Carlo simulations using the SSA developed by Gillespie [45] , [46] . In contrast to the deterministic framework in which the state of the system is defined by the concentrations of all species, which vary continuously with time, the state of the system in the stochastic framework is defined by the number of occurrences of each species and these change discretely whenever one reaction is executed. The likelihood that a particular reaction is executed is proportional to its rate constant and the numbers of its reactants. Using the SSA, we simulated the time evolution of the excess helical sense as a function of added 'sergeant' at each temperature using the appropriate thermodynamic values obtained by analysis of the single-component systems (Methods) and a temperature-independent mismatch penalty, , of −0.5 kJ mol −1 . From each of these simulations, where 500,000 molecules were followed for 20,000,000,000 reactions, the corresponding monomer and polymer concentrations were calculated by averaging over the last quarter of the simulation, in which these concentrations fluctuated around their equilibrium values. Figure 6a (right axis) shows that the computed excess helical sense at equilibrium describes the experimental titrations remarkably well for all temperatures considered. Indeed, the simulations correctly predict that at high temperatures, the excess helical sense reaches a maximum for low fractions of ( R )- 1 . The cause of this counterintuitive effect is understood by analysing the simulations in more detail. Figure 6c displays the calculated total monomer concentration, together with the total material in P - and M -type helical aggregates, as a function of added 'sergeant' at a temperature of 337 K. Whereas addition of <15% of 'sergeant' results in the expected decrease in concentration of supramolecular polymers with the wrong helical sense ( M -type) and increase in concentration of P -type helical aggregates; addition of >15% of ( R )- 1 results in a notable decrease in the total material present in P -type aggregates accompanied by a concomitant increase in the total concentration of monomers. The origin of this effect can be found in the lower T e of chiral homopolymers ( Supplementary Fig. S4 ), which is clearly visible in the measurements ( Fig. 6b ) and the simulated melting curves ( Fig. 6d ). Therefore, at high temperatures and high fraction of 'sergeant', partial melting of supramolecular copolymers occurs. This effect is most clearly visible when the sergeants-and-soldiers titrations are performed at a temperature between the T e of the homoaggregates consisting of ( A )- 2 and ( R )- 1 (347 K), where complete melting of the hetero-aggregates occurs for values of χ >80% ( Supplementary Fig. S5 ). We have presented a new model to describe chiral amplification that takes into account the coupling between the growth of the supramolecular polymer and the monomer pool in two-component self-assembling systems. We have shown that the thermodynamic equilibrium for the model can be calculated using two distinct methodologies, that is, either by solving the mass-balance equations or by following the kinetics of the system using stochastic simulation. Although the majority-rules principle has been analysed using a mass-balance approach and the sergeants-and-soldiers principle using a stochastic simulation approach, both methods can be used for both systems, providing the same results. Both methodologies, however, have their own advantages. The main advantage of the mass-balance method is that the concentrations at thermodynamic equilibrium can be obtained very efficiently. Moreover, this approach can be used to derive explicit formulas, like the expression for the critical ee. 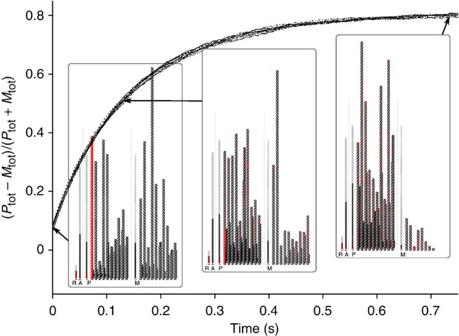Figure 7: Sergeants-and-soldiers chiral amplification kinetics. Simulated chiral amplification kinetics evolving via the sergeants-and-soldiers principle upon titration of a solution of (R)-1in heptane (χ=10%) to a solution of (A)-2in heptane (χ=90%) at a total concentration of 2.1×10−5M and a temperature of 337 K. Nine lines from different simulations, using 5,000,000 molecules, are shown. The insets show snapshots of a movie that was constructed from the time-dependent output of such simulations using 10,000 molecules. On mixing of chiral (R)-1as aggregates (red), monomer dissociation results in incorporation of chiral monomers in achiralP- andM-type stacks (black) eventually leading to a breakdown of theM-type aggregates. Chiral amplification was quantified as (Ptot−Mtot)/(Ptot+Mtot), in whichPtotandMtotrepresent the concentration of BTA molecules inP- andM-type aggregates, respectively. The full movies are available in theSupplementary Information. Advantage of the computationally much more demanding stochastic simulation approach is that also the kinetics can be followed, as is shown in Figure 7 for the sergeants-and-soldiers chiral amplification kinetics, and that the output of the simulations can be visualized as movies. Supplementary Movies 1 , 2 , 3 (see also Supplementary Fig. S6 ) demonstrate the simulation approach and nicely illustrate the difference between isodesmic and cooperative supramolecular polymerizations. Supplementary Movies 4 and 5 (see also Supplementary Fig. S7 ) demonstrate the majority-rules principle and the influence of the mismatch penalty, whereas Supplementary Movies 6 and 7 (see also Supplementary Fig. S8 ) focus on the sergeants-and-soldiers principle. Such movies provide the chemist with a novel visual tool to enhance their understanding of molecular events in multi-component mixtures of self-assembling molecules. The use of such visual tools will become increasingly important for chemists as the complexity of self-assembling systems is ever increasing. Figure 7: Sergeants-and-soldiers chiral amplification kinetics. Simulated chiral amplification kinetics evolving via the sergeants-and-soldiers principle upon titration of a solution of ( R )- 1 in heptane ( χ =10%) to a solution of ( A )- 2 in heptane ( χ =90%) at a total concentration of 2.1×10 −5 M and a temperature of 337 K. Nine lines from different simulations, using 5,000,000 molecules, are shown. The insets show snapshots of a movie that was constructed from the time-dependent output of such simulations using 10,000 molecules. On mixing of chiral ( R )- 1 as aggregates (red), monomer dissociation results in incorporation of chiral monomers in achiral P - and M -type stacks (black) eventually leading to a breakdown of the M -type aggregates. Chiral amplification was quantified as ( P tot − M tot )/( P tot + M tot ), in which P tot and M tot represent the concentration of BTA molecules in P - and M -type aggregates, respectively. The full movies are available in the Supplementary Information . Full size image In conclusion, we have analysed mathematical models for chiral amplification in cooperative supramolecular copolymerizations that take into account the coupling between the growth of the supramolecular polymer and the monomer pool. We have shown that the thermodynamic equilibrium can be calculated by solving mass-balance equations or by following the kinetics of the system using stochastic simulation. Both techniques were used to give new insight into two different examples of chiral amplification in two-component mixtures, that is, the majority-rules and the sergeants-and-soldiers effect. Using a common reaction scheme, the models perfectly fit both effects over a wide range of temperatures, concentrations and ratios of monomers. Moreover, we have shown that chiral amplification evolving via the majority-rules principle leads to an asymmetric depletion of the enantiomerically related monomer pool. Current experimental and theoretical work is aimed at a three-component self-assembling BTA system, in which two enantiomerically related components are able to undergo racemization in the presence of a catalytic amount of non-racemizable BTA. Such systems are expected to undergo chiral symmetry breaking and therefore may prove valuable in the field of asymmetric synthesis. Mass-balance model for the majority-rules principle The mass-balance model is based on the principle of detailed balance, which states that in thermodynamic equilibrium also each individual reaction is in equilibrium. For instance, for the formation of the P -type nucleus , which has an equilibrium constant σK E1 , this implies that . Similarly for the reaction ( P -type), with equilibrium constant K E2 , it holds that . In general, the concentration of an arbitrary P -type polymer of length i + j that contains i molecules R and j molecules S is given by . Since there are different types of polymers of length ℓ with i molecules R , the concentration of P -type polymers with length ℓ is given by where is the elongation factor for P -type polymers, and we used the binomial theorem in the last step. Clearly g P <1, otherwise the system would contain an infinite number of molecules. The total amount of molecules in all P -type polymers is then given by where we used the identity for | a |<1. Next, we consider the R molecules in P -type polymers. The amount of R molecules in P -type polymers of length ℓ is given by The total amount of R molecules in all P -type polymers is given by summing this expression over all ℓ ≥2, which yields where we have used the identity for | a |<1. Similarly, the amount of R molecules in M -type polymers of length ℓ is found to be where is the elongation factor for M -type polymers. Also g M must be <1 for a finite system. For the total amount of R molecules in all M -type polymers, we now obtain Each R molecule is a free monomer, or part of a P -type polymer or part of an M -type polymer. This mass-balance condition for R molecules gives > , which implies In the same way, we can compute the amount of S molecules in P - and M -type polymers. The mass-balance condition for S molecules finally gives The expressions (14) and (15) form a nonlinear system of equations with the monomer concentrations r and s as unknowns. Facilitated by the introduction of two new variables x and y instead of r and s , with we solved these coupled equations numerically using Matlab. Once the free-monomer concentrations r and s are known, the total amounts of molecules in P - and M -type polymers can easily be computed from equation (13) and a similar expression for M tot . Repeating this procedure for various temperatures and/or for various combinations of r tot and s tot leads to Figures 4a,c,d and 5a,b . Derivation of the critical ee The elongation factor g P describes how the concentration of P -type polymers of length ℓ depends on ℓ . Clearly g P <1, otherwise the total material in P -type polymers will be infinite. The same holds for the elongation factor g M . We first consider the case ee=0, which means r tot = s tot = c tot /2. Since the total concentration c tot is assumed to be large, most of the material must be in P -type and M -type polymers. That is only possible if both elongation factors are ~1. The equations g P =1 and g M =1 have as solution r = s = 1/( K E1 + K E2 ). That is indeed the value of the monomer concentrations r and s at ee=0. The numerically found solution shown in Figure 4c implies that r and s have approximately this value for all ee up to the critical value ee cr . To compute ee cr , we first rewrite the mass-balance equations as Substitution of r = s = 1/( K E1 + K E2 ) and g P = g M =1 in these equations leads to This is a linear system of equations, with P tot and M tot as unknowns. The solution, written as a function of ee = ( r tot − s tot ) / c tot is given by Note that P tot increases linearly with ee and M tot decreases linearly with ee, as can be seen in the left part of Figure 4c . The decrease of M tot is possible until it vanishes, which happens if This is the expression for the critical value of the ee. Gillespie simulation of the sergeants-and-soldiers principle In contrast to the deterministic framework in which the state of the system is defined by the concentration of each species, which vary continuously with time, the state of the system in the stochastic Gillespie framework [45] is defined by the number of occurrences of each species, and these change discretely whenever one of the reactions is executed. In the case of a supramolecular polymerization of a single monomer type X, as described by the reactions in equation (1), the current state of the system is given by the number of monomers and the numbers of polymers and their lengths. Given these numbers of monomers and polymers and the reaction rates, the probabilities of all possible reactions can be calculated. These possible reactions are dimerization, that is, the formation of a new oligomer from two monomers, and the addition or dissociation of one monomer to/from one of the polymers present. The system that we use to study the supramolecular polymerization consists of N molecules in a box with volume V . As initial configuration for the simulations, all N molecules are present as monomers. The initial concentration of monomer c tot thus equals N / V . During the simulation, new supramolecular polymers can be created by dimerization of two monomers. These polymers can then grow and shrink by the addition/dissociation of monomers. At each iteration of the simulation, the probabilities of all possible reactions are calculated and one reaction is selected proportional to these probabilities and is executed. After a reaction has been selected, products are stoichiometrically incremented, reactants are decremented and the time by which the system advances is determined by randomly drawing a number from an exponential distribution with as parameter the sum of all reaction propensities. In the Supplementary Information, a number of simulations on single-component isodesmic and cooperative supramolecular polymerizations are shown ( Supplementary Fig. S6 ). In the case of supramolecular copolymerization, two different monomer types are present. For such two-component systems, the number of possible species becomes extremely large. Therefore, in our simulations, species and reactions are introduced into the simulation programme only when they become needed, and removed whenever they become no longer needed. Although with the addition of the second component, we have to keep track of an increased number of reaction events ( Fig. 3 ), the simulation method remains exactly the same. I.e., we keep track on the current state (number of monomers and all polymers), calculate all reaction probabilities and randomly select one according to this probability distribution. We have assumed a diffusion-controlled association rate constant (10 10 M −1 s −1 ), both for the dimerization reactions and for the monomer additions to aggregates, which is independent of the monomer type, aggregate length and aggregate handedness [47] , [48] . After fixing all association rate constants to this value, all monomer dissociation rate constants of the various P - and M -type assemblies can be calculated from equations (2,3,4,5) using the appropriate thermodynamic parameters. Thermodynamic parameters The thermodynamic parameters used have been determined from analysis of single-component systems as described in the Supplementary Methods . Analysis of the single-component systems, with MCH as a solvent (as was used for the majority-rules experiments), yields for the entropy increment Δ S 0 =−0.128 kJ mol −1 K−1 and for the enthalpy increments = −72 kJ mol −1 and = −30 kJ mol −1 . Analysis of single-component systems, with heptane as a solvent (as was used for the sergeants-and-soldiers experiments), yields for the chiral ( R )- 1 entropy increment Δ S 0 =−0.1015 kJ/ mol −1 K−1 and for the enthalpy increments = −66 kJ mol −1 and = −35 kJ mol −1 , and for the achiral ( A )- 2 entropy increment Δ S 0,A =−0.1255 kJ mol −1 K −1 , and for the enthalpy increments = −75 kJ mol −1 and = −27 kJ mol −1 . How to cite this article: Markvoort, A. J. et al . Theoretical models of nonlinear effects in two-component cooperative supramolecular copolymerizations. Nat. Commun. 2:509 doi: 10.1038/ncomms1517 (2011).